Parkinson's disease induced pluripotent stem cells with triplication of the α-synuclein locus A major barrier to research on Parkinson's disease is inaccessibility of diseased tissue for study. One solution is to derive induced pluripotent stem cells from patients and differentiate them into neurons affected by disease. Triplication of SNCA , encoding α-synuclein, causes a fully penetrant, aggressive form of Parkinson's disease with dementia. α-Synuclein dysfunction is the critical pathogenic event in Parkinson's disease, multiple system atrophy and dementia with Lewy bodies. Here we produce multiple induced pluripotent stem cell lines from an SNCA triplication patient and an unaffected first-degree relative. When these cells are differentiated into midbrain dopaminergic neurons, those from the patient produce double the amount of α-synuclein protein as neurons from the unaffected relative, precisely recapitulating the cause of Parkinson's disease in these individuals. This model represents a new experimental system to identify compounds that reduce levels of α-synuclein, and to investigate the mechanistic basis of neurodegeneration caused by α-synuclein dysfunction. Parkinson's disease (PD) is the most common neurodegenerative movement disorder [1] . The pathological hallmark is loss of midbrain dopaminergic neurons in the substantia nigra pars compacta, and abnormal fibrillar cytoplasmic inclusions called Lewy bodies are typically deposited in surviving neurons throughout the brain [2] . It is unclear why neurons degenerate in PD, but clues have been provided through studying the underlying genetics of the disorder [3] . SNCA , encoding α-synuclein, was the first gene linked to familial PD [4] , and α-synuclein is the principal protein constituent of Lewy bodies [5] . Furthermore, multiplications of the SNCA gene cause familial PD, with several duplication and triplication kindreds described [6] , [7] . Finally, multiple genome-wide association studies have established that variation at the SNCA locus is the most significant genetic risk factor for sporadic PD [8] , [9] . A meta-analysis of this data has found further association 5′ of SNCA , suggesting variation in promoter/enhancer regions may modulate expression of SNCA [10] . Taken together, α-synuclein clearly has a central role in PD pathogenesis, but modelling how it leads to neuronal death in PD has been difficult, in part, owing to the inaccessibility of diseased neurons from patients. Moreover, by the time PD manifests clinically, most of these cells have already been lost [11] . Transgenic models of α-synuclein have illuminated pathogenic processes operating in PD [12] , [13] , but have not fully replicated the phenotype of the human disease [14] . Existing primary and tumour cell models also have major drawbacks. Primary neuronal cultures from mice or rats are difficult to maintain in vitro and do not self-renew, and wild-type animals have an amino acid at position 53 of α-synuclein that, in humans, causes PD [15] . Transformed cell lines can be genetically manipulated for studying proteins of interest, but these cells carry mutations in genes involved in apoptosis and chromosomal rearrangements that can disrupt cell signalling pathways, and are phenotypically different from the cells affected by PD, all of which limits their use as a model system [16] , [17] . Many of the existing cellular models rely on poorly controlled overexpression of transgenes, a particular drawback when modelling a disease where subtle alteration of gene dosage is critical [18] . A potential solution is to utilize reprogamming technology to generate disease-specific induced pluripotent stem cells (iPSCs) [19] . iPSCs derived from patients with PD can then be differentiated to midbrain dopaminergic neurons for disease modelling. Generation of iPSCs from individuals with sporadic PD has been reported [20] , [21] . Given the long latency and variability of disease progression, and that epigenetic modifications are erased during the process of generating iPSCs, it is unclear whether such patient-derived cells can recapitulate pathogenesis in cell culture [22] , [23] . More recently, an iPSC model of PD caused by homozygous G2019S mutation of LRRK2 has been reported [24] . However, LRRK2 mutations have incomplete penetrance, even when homozygous [25] . To overcome these difficulties, we sought to develop an iPSC-based model of PD with fibroblasts from an affected member of the Iowa kindred carrying a triplication of the SNCA locus, to serve as a model of the sporadic disorder. SNCA triplication results in four copies of the SNCA gene and a doubling of messenger RNA and protein expression [6] , [26] , [27] . This causes early onset, rapidly progressive form of PD that is fully penetrant, circumventing the influence of epigenetic changes, and maximizing the chances of an iPSC model developing a disease phenotype in vitro . We asked whether it would be possible to recapitulate α-synuclein doubling in patient-derived iPSCs differentiated into dopaminergic neurons. If so, the α-synuclein doubling would have the important benefit of providing a measurable biomarker, which could be used as a diagnostic test to validate the model, and provide a platform for drug screening and mechanistic experiments. We describe the generation of sets of iPSC lines from a patient with triplication of SNCA , and an unaffected first-degree relative, serving as a control with a similar genetic background, to minimize phenotypic differences not due to the triplication. Once differentiated into cultures enriched for midbrain dopaminergic neurons, a twofold increase in expression of SNCA was demonstrated in patient-derived cells, when compared with control cells that had undergone neural differentiation with equivalent efficiency. A major source of variability identified in this work was iPSC clonal variation, which partly contributed to differences in efficiency of differentiation. This emphasizes the need to generate multiple iPSC lines from each individual involved in a study of this nature, to identify clones with capacity to differentiate into cells of interest, and also to take steps to compare neuronal cultures with equivalent differentiation efficiency. PD fibroblasts do not express α-synuclein Muenter and co-workers reported the original description of the Iowan kindred, with a long family history of early-onset Parkinsonism and dementia [28] . Subsequently, a triplication of a region on Chr4q22 encompassing the SNCA locus was identified in this kindred [6] . Fibroblast cultures were established from dermal biopsies provided by a female member with PD and an unaffected first-degree relative. For clinical description and video documentation of the patient, see case 9-60 in Gwinn et al . [29] We refer to patient-derived cells as AST (alpha-synuclein triplication) and relative-derived cells as NAS (normal alpha-synuclein). Neither AST nor NAS fibroblasts expressed detectable levels of α-synuclein protein ( Fig. 1a ). This suggests that the triplication does not result in significant ectopic expression of this pre-synaptic protein. 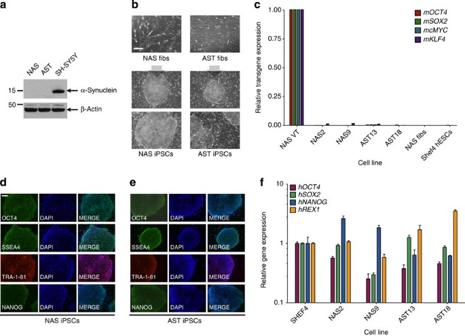Figure 1: Multiple iPSC lines derived from a PD patient withSNCAtriplication and an unaffected relative exhibit hallmarks of pluripotency. (a) Western blot analysis of AST and NAS fibroblasts confirms a lack of α-synuclein protein. Lysate of SH-SY5Y neuroblastoma cells transfected with an α-synuclein expressing plasmid was used as a positive control, and β-actin as a loading control. (b) Phase contrast images of AST and NAS fibroblasts andde novoiPSC colonies on SNL feeder cells at day 20 post-viral transduction. Scale bar, 100 μm. (c) Quantitative RT–PCR for retroviral transgene expression of the four reprogramming factors (Oct4,Sox2,c-Myc,Klf4). Expression in iPSC lines was normalized to transgene expression of NAS fibroblasts 3 days post-viral transduction (NAS VT). Also shown are negative controls: untransduced fibroblasts (NAS fibs) and human ESCs (Shef4 hESC). (d, e) Representative iPSC colonies derived from NAS fibroblasts (d) and AST fibroblasts (e) stained positive for the pluripotency markers OCT4, SSEA4, TRA-1-81 and NANOG. Scale bar, 100 μm. (f) Endogenous expression ofOCT4,SOX2,NANOGandREX1in two AST and two NAS iPSC lines, normalized to expression in human ESCs (Shef4), found a similar expression profile in all lines examined. Expression of these genes was absent in human fibroblasts (not shown). Error bars represent standard deviation of technical replicates,n=3. Figure 1: Multiple iPSC lines derived from a PD patient with SNCA triplication and an unaffected relative exhibit hallmarks of pluripotency. ( a ) Western blot analysis of AST and NAS fibroblasts confirms a lack of α-synuclein protein. Lysate of SH-SY5Y neuroblastoma cells transfected with an α-synuclein expressing plasmid was used as a positive control, and β-actin as a loading control. ( b ) Phase contrast images of AST and NAS fibroblasts and de novo iPSC colonies on SNL feeder cells at day 20 post-viral transduction. Scale bar, 100 μm. ( c ) Quantitative RT–PCR for retroviral transgene expression of the four reprogramming factors ( Oct4 , Sox2 , c-Myc , Klf4 ). Expression in iPSC lines was normalized to transgene expression of NAS fibroblasts 3 days post-viral transduction (NAS VT). Also shown are negative controls: untransduced fibroblasts (NAS fibs) and human ESCs (Shef4 hESC). ( d, e ) Representative iPSC colonies derived from NAS fibroblasts ( d ) and AST fibroblasts ( e ) stained positive for the pluripotency markers OCT4, SSEA4, TRA-1-81 and NANOG. Scale bar, 100 μm. ( f ) Endogenous expression of OCT4 , SOX2 , NANOG and REX1 in two AST and two NAS iPSC lines, normalized to expression in human ESCs (Shef4), found a similar expression profile in all lines examined. Expression of these genes was absent in human fibroblasts (not shown). Error bars represent standard deviation of technical replicates, n =3. Full size image iPSC generation and characterization To generate iPSCs, fibroblasts were virally transduced with four reprogramming factors [19] . Figure 1b depicts fibroblasts and primary iPSC colonies at day 20 post-viral transduction. A total of 30 AST and 10 NAS iPSC lines were established. Cell lines with the strongest retroviral silencing have been shown to differentiate more efficiently and is indicative of complete reprogramming [30] . Therefore, all lines were examined for transgene silencing relative to fibroblasts 3 days post-viral transduction (acting as a positive control). The cell lines with the lowest levels of transgene expression were chosen for further analysis ( Fig. 1c ). All chosen iPSC lines exhibited good hESC colony morphology and growth characteristics, and have been passaged more than 35 times, with more than 6 months in continual culture. Colonies from NAS and AST iPSC lines demonstrated robust expression of the pluripotency markers OCT4, SSEA4, TRA-1-81 and NANOG ( Fig. 1d, e ). Endogenous expression of the pluripotency genes OCT4 , SOX2 , NANOG and REX1 was reactivated in all iPSC lines examined ( Fig. 1f ). The OCT4 and SOX2 primers do not recognize the mouse Oct4 and Sox2 transgenes used to reprogram the cells. No significant differences between AST and NAS iPSC lines were observed with respect to expression of key pluripotency genes. Triplication status and chromosomal integrity SNCA gene dosage was re-examined in the AST iPSC lines to confirm they retained the triplication: genomic qPCR for SNCA exons 1 and 4 confirmed that AST iPSC lines had twice as many SNCA alleles as NAS iPSC lines ( Fig. 2a ). Genomic DNA samples from the two participants, the two fibroblast lines, four iPSC lines, and differentiated neurons were further analysed on genome-wide SNP arrays. This analysis confirmed that those samples derived from the unaffected relative were normal at Chr4q22 ( Fig. 2b ) whereas the triplicated region was retained intact in all samples derived from the patient ( Fig. 2c ). We were able to refine the triplication region further [6] and determined the size to be 1.505 Mb ( Fig. 2d ). We were also able to survey the rest of the genome for chromosomal integrity in these cell lines. Two PD iPSC lines (AST13 and AST18) and one control iPSC line (NAS2) did not acquire any chromosomal aberrations after more than 25 passages. However one control iPSC line, NAS9, contained a duplication of a large part of chromosome 5q, an extended run of homozygosity in chromosome 12q, and a small deletion at the end of chromosome 4q ( Fig. 2e ). Chromosomal abnormalities of this nature are consistent with published reports of iPSCs where this has been specifically examined [31] . However, such analysis has not been reported in the iPSC disease models published so far. This SNP data also confirmed that AST and NAS iPSCs and neurons were indeed derived from the PD patient and unaffected relative, respectively ( Table 1 ) [32] . 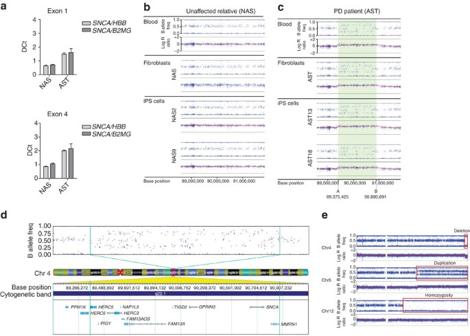Figure 2: Triplication region is maintained in patient-derived fibroblasts and iPSCs. (a) Quantitative genomic PCR forSNCAexons 1 and 4 demonstrates doubling of gene dosage in patient-derived AST iPSC lines when compared with NAS iPSC lines. Representative data shown.SNCAwas normalized to β-globin (HBB) and β2-microglobulin (B2MG). (b) SNP profiles of chromosome 4q22 in DNA from unaffected relative blood, fibroblasts and iPSCs demonstrates that this region is normal. (c) The same region analysed in DNA from patient blood, fibroblasts and iPSCs confirms that the triplication region is present and is retained during reprogramming. (d) The triplication region is defined as chr4:89,375,425 to 90,880,891, spanning the following genes:HERC5,PIGY,HERC3,NAP1L5,FAM13AOS,FAM13A,TIGD2,GPRIN3,SNCAandMMRN1.LOC644248is also in the triplication region but not yet defined by RefSeq. (e) Genome-wide SNP analysis of NAS9 iPSCs identified the following chromosomal abnormalities: a small deletion at the end of Chr4q, a duplication of part of Chr5q and an extended run of homozygosity occupying most of Chr12q. Figure 2: Triplication region is maintained in patient-derived fibroblasts and iPSCs. ( a ) Quantitative genomic PCR for SNCA exons 1 and 4 demonstrates doubling of gene dosage in patient-derived AST iPSC lines when compared with NAS iPSC lines. Representative data shown. SNCA was normalized to β-globin ( HBB ) and β2-microglobulin ( B2MG ). ( b ) SNP profiles of chromosome 4q22 in DNA from unaffected relative blood, fibroblasts and iPSCs demonstrates that this region is normal. ( c ) The same region analysed in DNA from patient blood, fibroblasts and iPSCs confirms that the triplication region is present and is retained during reprogramming. ( d ) The triplication region is defined as chr4:89,375,425 to 90,880,891, spanning the following genes: HERC5 , PIGY , HERC3 , NAP1L5 , FAM13AOS , FAM13A , TIGD2 , GPRIN3 , SNCA and MMRN1 . LOC644248 is also in the triplication region but not yet defined by RefSeq. ( e ) Genome-wide SNP analysis of NAS9 iPSCs identified the following chromosomal abnormalities: a small deletion at the end of Chr4q, a duplication of part of Chr5q and an extended run of homozygosity occupying most of Chr12q. Full size image Table 1 Pi-hat analysis confirms origin of iPSC lines and neurons. Full size table Directed differentiation to dopaminergic neurons We used a feeder-free monolayer culture method of inducing neural differentiation under defined conditions, via dual inhibition of SMAD signalling [33] . This approach combines Noggin (an inhibitor of BMP4) and SB431542 (an inhibitor of Lefty/Activin/TGFβ pathways) to achieve robust neural differentiation. Here we have also added Dorsomorphin (a chemical BMP inhibitor) as a partial substitute for Noggin, to improve efficiency and reduce costs [34] . The dual SMAD inhibition protocol has been employed to generate floor plate tissue from human ESCs [35] . Fasano and co-workers demonstrated directed differentiation of human ESCs into floor plate tissue via initial dual SMAD inhibition in conjunction with early high-dose sonic hedgehog (SHH) signalling [35] . We commenced neural differentiation with dual SMAD inhibition for 1 day, followed by SHH, WNT1 and Dkk1 blocking antibody treatment. After 9 days of floor plate differentiation, the protocol was switched to promote maturation of midbrain dopaminergic neurons from neural progenitors derived from human ESCs ( Fig. 3a ) [36] . 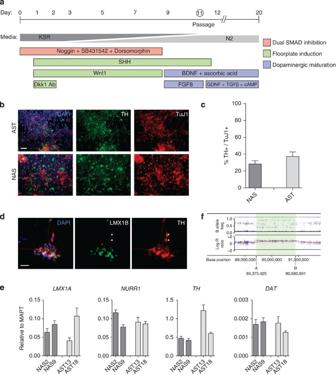Figure 3: Patient and control iPSC lines differentiate efficiently into midbrain dopaminergic neurons. (a) Schematic of the dual SMAD inhibition/floor plate protocol used to promote differentiation of iPSCs to a midbrain dopaminergic fate. (b) Immunocytochemistry of neuralized AST and NAS iPSCs for TuJ1 (red) and tyrosine hydroxylase (TH – green) shows robust differentiation into dopaminergic neurons. Scale bar, 100 μm. (c) Counts of TH+ neurons, expressed as a percentage of TuJ1+ neurons (n=1955 total), found no significant difference in efficiency of dopaminergic differentiation between AST and NAS iPSCs. Error bars represent standard deviation of biological replicates,n=3. (d) LMX1B (green) is expressed in the majority of TH+ (red) neurons (>80%). A minority of TH+ cells are negative for LMX1B (arrowheads). Scale bar, 100 μm. (e) Quantitative RT–PCR analysis for midbrain dopaminergic neural markers (LMX1A,NURR1,THandDAT) in AST and NAS neuronal cultures. To control for efficiency of neuralization we normalized expression to the pan-neuronal marker MAPT. Error bars represent standard deviation of technical replicates,n=3. (f) SNP analysis of AST-derived neurons confirms that the triplication region is retained intact following neuronal differentiation. Figure 3: Patient and control iPSC lines differentiate efficiently into midbrain dopaminergic neurons. ( a ) Schematic of the dual SMAD inhibition/floor plate protocol used to promote differentiation of iPSCs to a midbrain dopaminergic fate. ( b ) Immunocytochemistry of neuralized AST and NAS iPSCs for TuJ1 (red) and tyrosine hydroxylase (TH – green) shows robust differentiation into dopaminergic neurons. Scale bar, 100 μm. ( c ) Counts of TH+ neurons, expressed as a percentage of TuJ1+ neurons ( n =1955 total), found no significant difference in efficiency of dopaminergic differentiation between AST and NAS iPSCs. Error bars represent standard deviation of biological replicates, n =3. ( d ) LMX1B (green) is expressed in the majority of TH+ (red) neurons (>80%). A minority of TH+ cells are negative for LMX1B (arrowheads). Scale bar, 100 μm. ( e ) Quantitative RT–PCR analysis for midbrain dopaminergic neural markers ( LMX1A , NURR1 , TH and DAT ) in AST and NAS neuronal cultures. To control for efficiency of neuralization we normalized expression to the pan-neuronal marker MAPT. Error bars represent standard deviation of technical replicates, n =3. ( f ) SNP analysis of AST-derived neurons confirms that the triplication region is retained intact following neuronal differentiation. Full size image Eight AST and six NAS iPSC lines were subjected to the floor plate-dopaminergic differentiation protocol. Five AST lines and four NAS lines produced viable neurons that could be analysed. After 20 to 31 days, differentiated iPSCs were examined for tyrosine hydroxylase (TH - the rate-limiting enzyme in the biosynthetic pathway to dopamine, used as a marker of dopaminergic neuronal identity) and neuron-specific class III β-tubulin (TuJ1 - used as a marker of pan-neuronal identity) and all showed robust expression of these markers ( Fig. 3b ). We performed blind cell counts on micrographs fluorescently labelled for TH and TuJ1, and found that AST iPSCs yielded 37% (s.d. 5) TH-positive cells as a proportion of TuJ1-positive cells whereas NAS iPSCs yielded 28% (s.d. 4), which is not significantly different ( Fig. 3c ). We confirmed the midbrain identity of these TH-positive neurons by co-immunolabelling with the ventral midbrain marker LMX1B ( Fig. 3d ) [37] . To further confirm their midbrain dopaminergic identity, we performed expression analysis of LMX1A , NURR1 , TH and DAT ( Fig. 3e ). We observed a range of expression of these factors that was not linked to genotype. This may reflect clonal variation or efficiency of neuralization that has been previously observed in iPSCs [38] . Genome-wide SNP analysis of AST iPSC-derived neuronal cultures confirmed that the triplication region had remained intact during differentiation ( Fig. 3f ). α-Synuclein protein could be detected in all iPSC-derived neuronal cultures ( Fig. 4a, b ). We observed considerable heterogeneity of expression of α-synuclein that may reflect different neuronal subtypes or different stages of neuronal maturity [39] . However, α-synuclein was found to be expressed in all TuJ1+ cells. In contrast, it was not detectable in fibroblasts by immunocytochemistry or western ( Fig. 1a ). 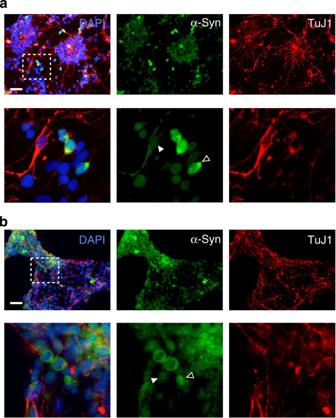Figure 4: Expression of α-synuclein in iPSC-derived neuronal cultures is heterogeneous. Expression of α-synuclein was observed in all TuJ1+ neurons derived from AST (a) and NAS (b) iPSCs. The majority of cells expressed low levels of α-synuclein (filled arrowheads) whereas 3–7% of TuJ1+ cells expressed a high level of protein (open arrowheads). Scale bar, 100 μm upper panels, 400 μm lower panels. Figure 4: Expression of α-synuclein in iPSC-derived neuronal cultures is heterogeneous. Expression of α-synuclein was observed in all TuJ1+ neurons derived from AST ( a ) and NAS ( b ) iPSCs. The majority of cells expressed low levels of α-synuclein (filled arrowheads) whereas 3–7% of TuJ1+ cells expressed a high level of protein (open arrowheads). Scale bar, 100 μm upper panels, 400 μm lower panels. Full size image Triplication gene set is over-expressed in AST neurons Gene expression profiling was carried out on the AST and NAS fibroblasts, four iPSC lines (AST13, AST18, NAS2, and NAS9) and eight neuronal cultures (Day 23 and Day 31 of the 4 iPSC lines). Principal component analysis (PCA) and hierarchical clustering found that the three groups of cell samples clustered separately, with the iPSCs most closely associated with a control human ESC line, Shef4 ( Fig. 5a, b ). Scatter plots comparing gene expression of iPSCs, and fibroblasts with that of human ESCs found that the overall expression profiles of human ESCs was more similar to iPSCs than the fibroblast cell lines ( Fig. 5c ). We were unable to detect any significant differences (at false discovery rate of 0.05) in genome-wide gene expression between human ESCs and iPSCs or NAS iPSCs as compared with AST iPSCs. To further confirm that our iPSC lines exhibited a pluripotent expression profile, we compared global gene expression with all publicly available hESC gene expression data sets using the same platform. The resulting PCA plots demonstrate that the expression profiles of the iPSC lines described are indistinguishable from established hESC lines ( Fig. 5d ). Following the creation of a triplication gene set (defined as all genes within the triplication region, shown in Fig. 2d ), we used gene set enrichment analysis (GSEA) to demonstrate a highly significant enrichment (nominal P -value <0.0001) of this set within AST as compared with NAS neurons ( Fig. 5e ). Although we were also able to demonstrate significant enrichment (nominal P -value <0.05) of the triplication gene set in AST versus NAS iPSCs, no significant enrichment could be detected in AST versus NAS fibroblasts (nominal P -value=0.09). We estimated the statistical significance (nominal P value) of the enrichment score by using an empirical gene set-based permutation test procedure, as described in Subramanian et al . [40] Specifically, we observed that SNCA expression is elevated in AST compared with NAS iPSCs and was further increased when these cells were differentiated into neurons ( Fig. 5f ). Expression was not detected in fibroblasts. 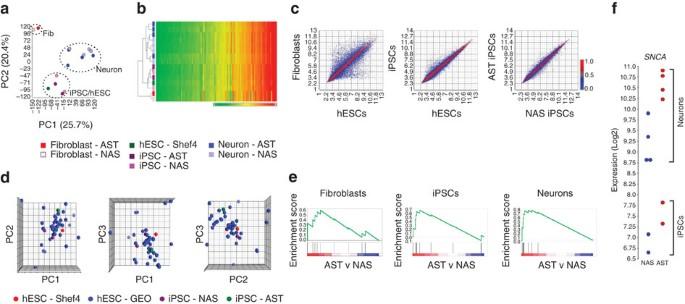Figure 5: Gene expression profiling finds that the triplication genes are significantly enriched in AST iPSC-derived neurons. Principle components analysis (a) and hierarchical clustering (b) shows that iPSCs cluster with hESCs, while fibroblasts and neurons cluster separately. There is no clear separation between AST and NAS-derived cells at this level of analysis. (c) Scatter plots demonstrate that global gene expression of iPSCs is more similar to hESCs than fibroblasts and there are no significant differences in global gene expression between AST and NAS iPSCs. (d) Multiple views of a three-dimensional PCA plot, following batch effect removal, comparing iPSC gene expression to all hESC data sets on the Affymetrix U133 Plus 2.0 platform that are publicly available (59 samples from 8 separate submissions). The iPSCs intermingle within the hESC landscape in all three dimensions. (e) Gene set enrichment analysis for the triplication genes shows significant enrichment in AST iPSCs (nominalP-value <0.05) and neurons (nominalP-value <0.0001) but not fibroblasts (nominalP-value=0.09). Enrichment scoreP-values are estimated by using an empirical gene set-based permutation test procedure40. (f)SNCAexpression is higher in AST-derived iPSCs and neurons than in equivalent cells from NAS. Figure 5: Gene expression profiling finds that the triplication genes are significantly enriched in AST iPSC-derived neurons. Principle components analysis ( a ) and hierarchical clustering ( b ) shows that iPSCs cluster with hESCs, while fibroblasts and neurons cluster separately. There is no clear separation between AST and NAS-derived cells at this level of analysis. ( c ) Scatter plots demonstrate that global gene expression of iPSCs is more similar to hESCs than fibroblasts and there are no significant differences in global gene expression between AST and NAS iPSCs. ( d ) Multiple views of a three-dimensional PCA plot, following batch effect removal, comparing iPSC gene expression to all hESC data sets on the Affymetrix U133 Plus 2.0 platform that are publicly available (59 samples from 8 separate submissions). The iPSCs intermingle within the hESC landscape in all three dimensions. ( e ) Gene set enrichment analysis for the triplication genes shows significant enrichment in AST iPSCs (nominal P -value <0.05) and neurons (nominal P -value <0.0001) but not fibroblasts (nominal P -value=0.09). Enrichment score P -values are estimated by using an empirical gene set-based permutation test procedure [40] . ( f ) SNCA expression is higher in AST-derived iPSCs and neurons than in equivalent cells from NAS. Full size image Assessment of neuralization and SNCA expression To determine whether AST neurons recapitulate the elevated SNCA expression observed in postmortem brain tissue in patients from this kindred, and to confirm the microarray results ( Fig. 5f ), we performed further neuronal differentiations and carried out quantitative RT–PCR analysis of SNCA . We found that AST-derived neurons expressed approximately double the quantity of SNCA mRNA as NAS-derived neurons, when controlling for efficiency of neuralization by normalizing to the pan-neuronal marker MAPT ( Fig. 6a ). SNCA has two paralogous genes, SNCB and SNCG , which respectively encode β- and γ-synuclein. All have been found in neuritic pathology in PD and dementia with Lewy bodies [41] . Wild-type β-synuclein inhibits α-synuclein aggregation in vitro and limits pathology due to human α-synuclein expression in transgenic mice, but can cause neurodegeneration when mutated [42] , [43] . In contrast, transgenic overexpression of wild-type γ-synuclein leads to neurodegeneration [44] . Overall, β-synuclein appears to be protective whereas γ-synuclein may exert its own toxicity. We observed that SNCG expression was significantly lower in AST neurons, suggesting a possible compensatory mechanism. No significant difference was observed in the expression of SNCB ( Fig. 6a ). 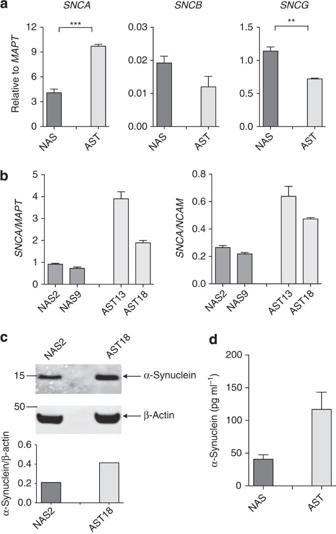Figure 6:SNCAexpression is doubled in selected iPSC lines when controlling for efficiency of neuralization. (a) RT–PCR data forSNCA,SNCBandSNCGshows that expression ofSNCAis significantly higher, andSNCGsignificantly lower, in AST iPSC-derived neurons when efficiency of neuralization is controlled for, by normalizing to expression of the pan-neuronal marker MAPT. Error bars represent standard deviation of technical replicates,n=3. ***P<0.0005; **P<0.005 (Student'st-test, unpaired, two-tailed). (b) Quantitative RT–PCR analysis ofSNCAexpression, normalized to pan-neuronal markers (NCAM,MAPT) to directly control for efficiency of differentiation, shows a twofold or greater increase inSNCAexpression in neurons derived from AST iPSCs. Error bars represent standard deviation of technical replicates,n=3. (c) Western blot analysis of Day 20 neuronal cultures showed that AST18 expressed double the amount of α-synuclein protein as NAS2, despite differentiating into neurons with the same efficiency. (d) ELISA detects significantly more α-synuclein in 48 h conditioned media from AST neuronal cultures than equivalently conditioned media from NAS neuronal cultures. Error bars represent standard deviation of biological replicates,n=2. Figure 6: SNCA expression is doubled in selected iPSC lines when controlling for efficiency of neuralization. ( a ) RT–PCR data for SNCA , SNCB and SNCG shows that expression of SNCA is significantly higher, and SNCG significantly lower, in AST iPSC-derived neurons when efficiency of neuralization is controlled for, by normalizing to expression of the pan-neuronal marker MAPT. Error bars represent standard deviation of technical replicates, n =3. *** P <0.0005; ** P <0.005 (Student's t -test, unpaired, two-tailed). ( b ) Quantitative RT–PCR analysis of SNCA expression, normalized to pan-neuronal markers ( NCAM , MAPT ) to directly control for efficiency of differentiation, shows a twofold or greater increase in SNCA expression in neurons derived from AST iPSCs. Error bars represent standard deviation of technical replicates, n =3. ( c ) Western blot analysis of Day 20 neuronal cultures showed that AST18 expressed double the amount of α-synuclein protein as NAS2, despite differentiating into neurons with the same efficiency. ( d ) ELISA detects significantly more α-synuclein in 48 h conditioned media from AST neuronal cultures than equivalently conditioned media from NAS neuronal cultures. Error bars represent standard deviation of biological replicates, n =2. Full size image To further probe the possibility of clonal variation, we investigated the level of expression of SNCA in multiple NAS and AST iPSC lines. AST13, AST18, NAS2 and NAS9 gave robust yields of neurons on repeated trials of neuralization. To control for heterogeneity of neuronal differentiation, we normalized SNCA expression to pan-neuronal markers ( MAPT and NCAM ). As for the dopaminergic markers ( Fig. 3e ), we observed some variation between lines, but we consistently found at least a doubling of SNCA expression in AST-derived neurons when compared with NAS-derived neurons ( Fig. 6b ). We next examined the level of α-synuclein protein expression in a pair of iPSC lines that differentiated with similar efficiency, AST18 and NAS2. A twofold increase in α-synuclein protein expression was observed in AST18 ( Fig. 6c ), which agreed with the difference in mRNA expression. Finally, we asked whether AST-derived neurons might release more α-synuclein into cell culture media than NAS-derived neurons, as this protein is known to be secreted by cells in culture [45] . We analysed 48 h conditioned media from several AST and NAS neuronal cultures and found significantly more α-synuclein released into the media from AST neurons ( Fig. 6d ). iPSC technology has the potential to revolutionize our understanding of PD, because it provides the opportunity to generate and study disease-affected cells directly from patients. This approach has already been used to generate cell models for several neurological conditions: amyotrophic lateral sclerosis, sporadic PD, spinal muscular atrophy and familial dysautonomia have all been described [21] , [46] , [47] , [48] . Here we describe iPSC lines with triplication of SNCA (AST), and lines from a non-affected first-degree relative (NAS). Both sets of iPSC lines were screened for retroviral transgene silencing, pluripotent marker expression, and differentiation efficiency in a floor plate-dopaminergic neuronal specification protocol. All of the lines derived from the patient fibroblasts have the SNCA triplication intact, as determined by PCR on genomic DNA, and confirmed in a subset of lines with genome-wide SNP analysis. Subsets of iPSC lines from the patient and unaffected relative have been successfully differentiated into dopaminergic neurons. These lines passed all criteria, and patient-derived neurons exhibited a doubling of SNCA mRNA expression and α-synuclein protein. We highlight a number of potential variables that must be considered when establishing an iPSC disease model. Variability between iPSC clones, variable responses to neural differentiation protocols, and heterogeneity of neural differentiation must all be taken into account when considering the validity and robustness of pluripotent cell lines used to model human diseases such as PD. These sources of variation have also been observed in other iPSC models [38] , [49] , [50] . Therefore it is an implicit requirement to generate several independent iPSC lines from each patient involved in a study of this nature, and to examine efficiency of neuralization for fair comparisons to be made [51] . As we expect each neuronally differentiated patient-derived iPSC clone to exhibit a doubling of SNCA expression, ours is a simple and stringent system for examining the robustness of the iPSC disease-modelling paradigm. The application of iPSC technology to modelling diseases such as PD, with long latency and involvement of epigenetic factors that could be erased during reprogramming, is challenging [22] . However, we chose a fully penetrant, early onset and rapidly progressive familial PD to offset these two potential problems as far as possible. Application of extrinsic agents, to stimulate oxidative stress for example, could be used to help accelerate development of a phenotype [52] . This has recently been performed to investigate LRRK2 mutant iPSCs [24] . PD iPSC models are systems in which the earliest pathogenic changes that lead to disease can be studied, rather than ones in which end-stage pathology of PD is observed. The triplicated SNCA iPSCs are well positioned for these studies due to the fully penetrant and early-onset phenotype in humans. This is important, because determining these earliest responses might provide a mechanism whereby the disease can be halted before it progresses, and, furthermore, those pathological changes that occur at later stages in the disease may be protective rather than toxic [53] . iPSCs carrying the SNCA triplication will also provide a valuable tool to investigate cell-to-cell propagation of pathology, being primed to develop disease [54] . These cells will also be of value in studying other synucleinopathies in vitro . Clinically, SNCA triplication can generate the full spectrum of the synucleinopathies, including progressive supranuclear palsy, multiple system atrophy and dementia with Lewy bodies, as well as PD [28] . Pathologically, cases can include glial deposition of α-synuclein reminiscent of the glial cytoplasmic inclusions found in multiple system atrophy [55] . The differentiation of AST and NAS lines towards an oligodendroglial fate may be informative about the cellular processes operating in this disorder [56] . In conclusion, we have derived a collection of iPSC lines from a PD patient with triplication of the α-synuclein locus, and an unaffected first-degree relative. This study demonstrates the potential of human dopaminergic neurons in vitro as a model for studying Parkinson's disease. It also highlights the inherent variation in iPSC clones, which makes the interpretation of these models challenging. However, this collection of disease and control iPSC lines will serve as an invaluable resource to study many of the unresolved questions in PD pathogenesis. Fibroblast cultures Dermal fibroblast cultures were isolated from a member of the Iowa kindred carrying a triplication of the SNCA locus and an unaffected member of the family without this mutation, following approval of the Royal Free research ethics committee, Royal Free Hospital, London, UK and informed consent from the husband of the patient (as next of kin) and the unaffected relative. Samples were designated anonymous identifiers following collection. Skin punch biopsies (forearm) were cultured in 5 cm 2 sterile Petri dishes at 37°C in 5% CO 2 in 2 ml DMEM supplemented with 10% fetal bovine serum, penicillin (50 U ml −1 ), and streptomycin (50 μg ml −1 ) until fibroblasts were seen to migrate from the skin explants. Media volume was increased by 0.5 ml every 2 days. When plates were confluent, fibroblasts were lifted from dishes by trypsinizing with TrypLE (Invitrogen) and transferred to 10 cm 2 dishes for culturing. The case fibroblast sample (cat no. ND27760) has been deposited at the Coriell Institute for Medical Research ( http://www.coriell.org/ ) and is freely available for research purposes. iPSC generation The four mouse reprogramming factors inserted into the pMXs vector backbone were obtained from Addgene (pMXs-cMyc #13375, pMXs-Klf4 #13370, pMXs-Oct4 #13366, pMXs-Sox2 #13367) [19] . These were transfected into Platinum-A cells (Cell Biolabs #RV-102) with Lipofectamine 2000 (Invitrogen) to package viral particles. Target fibroblasts (100,000 cells) were transduced with virus in the presence of 6 ng ml −1 polybrene (Millipore #Tr-1003-G) twice on consecutive days, then lifted with Accutase (Invitrogen) a day later and replated on irradiated SNL feeders (available from European Collection of Cell Cultures, ECACC). The day after replating, media was switched to hESC medium (KO-DMEM, 20% KSR, 2 mM l-glutamine, 1× non-essential amino acids, 50 μM 2-mercaptoethanol, 50 U ml −1 penicillin, 50 μg ml−1 streptomycin (all from Invitrogen), and 20 ng ml −1 FGF2 (Peprotech)) containing 0.5 mM valproate (Merck) [57] . Colonies were mechanically picked after ~20 days and maintained on SNL feeders in hESC medium without valproate. Established iPSC lines were maintained in hESC medium containing 10 ng ml −1 FGF2. Transgene silencing and marker gene expression RNA was obtained from separate iPSC lines using the RNeasy Plus kit (Qiagen) according to manufacturer's instructions. Complementary DNA was generated via Superscript III (Invitrogen), and qPCR reactions were carried out with SYBR Green (Qiagen) on a Lightcycler 480 (Roche), with primer pairs specific to mouse Oct4 , Sox2 , Klf4 and c-Myc . Results were normalized to human TBP using the comparative C(T) method [58] and compared with equivalent values determined from fibroblasts 3 days post-viral transduction (positive control), Shef4 human ES cells (negative control) and non-transduced human fibroblasts (negative control). cDNA was generated from neuralized iPSCs by the same method, and qPCR reactions were carried out with the Universal Probe Library system (Roche) and normalized to GAPDH or MAPT. All primers are described in Supplementary Table S1 . Immunocytochemistry Cells were fixed in 4% paraformaldehyde at room temperature, or 100% methanol at −20°C for 15 minutes, then blocked and permeabilized with blocking buffer (2% goat serum, 0.1% Triton-X in phosphate buffered saline) overnight at 4°C before probing with the following primary antibodies (overnight in goat blocking buffer at 4°C): OCT4 (Santa Cruz #5279, mouse IgG2b, 1:200), TRA 1-81 (Biolegend #330701, mouse IgMκ, 1:600), SSEA4 (DSHB, mouse IgG3κ, neat), NANOG (Abcam #ab21624, rabbit IgG, 1:1000), TuJ-1 (R&D systems #MAB1195, mouse IgG2A), TH (R&D systems #MAB1423 clone TH-2, mouse IgG1), LMX1B (Rabbit polyclonal from Dai et al . [37] , 1:2000) and α-synuclein (BD Transduction Laboratories #610787, mouse IgG1). Appropriate AlexaFluor-488 and AlexaFluor-596-labelled secondary antibodies (Molecular Probes) were used at 1:1000, along with DAPI counterstaining, before imaging with an Olympus IX51 inverted fluorescent microscope or Leica DM IRE2 confocal microscope. SNCA triplication screening Genomic DNA was obtained from individual cell lines using the DNA blood and tissue kit (Qiagen) according to manufacturer's instructions, including RNase A to remove contaminating RNA. Dosage of SNCA was then assessed with SYBR Green qPCR on a Rotorgene unit (Qiagen) using primers specific for exons 1 and 4 of SNCA and β2-microglobulin ( B2MG ) and β-globin ( HBB ) as diploid control genes ( Supplementary Table S1 ) [59] . Monolayer neuronal differentiation iPSC cultures were dissociated with Accutase (Invitrogen) to generate single-cell suspensions, then differentially plated on gelatin-coated plasticware for 1 h in hESC medium in the presence of ROCK inhibitor (Y27632, Ascent) to remove SNL feeders. The nonattached cells were resuspended in MEF-CM (R&D systems) with 10 ng ml −1 FGF2 (Peprotech) and plated on growth-factor reduced Matrigel (BD) at a density of 25,000 cells cm −2 and allowed to propagate in self-renewal conditions for 72 h or until 70–90% confluent, whereupon media was changed to KSR medium containing 50 ng ml −1 Noggin (Peprotech), 10 μM SB431542 (Tocris) and 2 μM Dorsomorphin (Tocris) for the first day, with the addition of 200 ng ml −1 SHH C24II (R&D Systems) and 50 ng ml −1 Wnt1 (Peprotech) for the second day onwards. Dkk1 blocking antibody (100 ng ml −1 , R&D Systems) was also added for the second day only. After 5 days, KSR medium containing these ligands was cross-tapered with N2B27 medium (Stem Cells) containing the same ligands over 7 days (75% KSR and 25% N2B27 first day, 50% of each third day, and 25% KSR with 75% N2B27 fifth day). Once established in N2B27 conditions, Wnt1, Noggin, SB431542 and Dorsomorphin were withdrawn whereas SHH was maintained, and 20 ng ml −1 BDNF (Peprotech), 0.2 mM ascorbic acid (Sigma) and 100 ng ml −1 FGF8 (Peprotech) were added. Three days later, cells were dissociated with Hank's buffered saline solution for 1 h at room temperature, and lifted mechanically, then replated en bloc on to poly-l-ornithine/laminin-coated plasticware. Neuronal maturation ensued with BDNF and ascorbic acid as before, supplemented with 10 ng ml −1 GDNF (Peprotech), 1 ng ml −1 TGFβ3 (Peprotech) and 0.5 mM dibutyryl-cAMP (Merck) for the next 7 days. After a total of 23–31 days, the resulting neuronal cultures were analysed by immunocytochemistry, qPCR and western blot. Protein analysis Fibroblast cells, neuronal cells differentiated from AST and NAS iPSCs and control SH-SY5Y cells were collected in radio immunoprecipitation buffer (Cell Signaling Technologies) and protein concentrations estimated by BCA assay (Thermo Scientific). Samples were diluted to equivalent protein concentration and then 20 μg denatured by the addition of 4× sample buffer (Invitrogen) supplemented with β-mercaptoethanol and boiled at 100°C for 10 min, loaded onto 12% Bis Tris Acrylamide gels (Invitrogen) and proteins separated by SDS–PAGE. Following transfer to cellulose or PVDF membrane, blots were probed for α-synuclein (BD Transduction#610787) and β-actin (Sigma-Aldrich #A1978) then imaged using either ECL (Pierce) and Kodak film, or the Odyssey imaging system (LiCor Biosciences). To quantify α-synuclein release by neurons, 48 h conditioned medium from 1 well of a 6-well plate was concentrated with Amicon Ultra-15 Centrifugal Filter Unit (Millipore). Released α-synuclein was assessed using an α-synuclein ELISA kit (USCN Life catalogue #E91222Hu) as per manufacturer's protocol. SNP microarray DNA was extracted from fibroblasts, iPSCs and neuralized iPSC lines using the DNeasy Blood and Tissue Kit (Qiagen) according to the manufacturer's instructions. DNA was quantified spectroscopically (NanoDrop, Thermo Scientific) and 4 μl of 50 ng μl −1 genomic DNA and whole-genome amplified DNA samples were marked on the Illumina Infinium Omni1-Quad BeadChip (Illumina) according to the manufacturer′s instructions. The BeadChips were scanned using an iScan (Illumina) with an AutoLoader (Illumina). GenomeStudio v.1.8.X (Illumina) was used for analysing the data and generating SNP calls. SNP calls were created using the HumanOmni1-Quad_v1-0_B cluster file provided by Illumina as a reference. Pi-hat analysis was performed with PLINK v1.07 ( http://pngu.mgh.harvard.edu/purcell/plink/ ) [60] . All SNP data was deposited in the GEO database under accession code GSE28366 . Gene expression microarray Total RNA was extracted from fibroblasts, iPSCs and neuralized iPSC lines using the RNeasy Plus kit (Qiagen), according to the manufacturer's instructions. Following the evaluation of RNA quality by capillary electrophoresis (Agilent 2100 Bioanalyzer and RNA 6000 Nano Kit, Agilent) 200 ng of total RNA was used as starting material for the cDNA preparation. All steps starting from the first and second strand cDNA synthesis, the in vitro transcription reaction to generate cRNA and the second round of cDNA synthesis were performed using the AmbionWT Expression Kit (Ambion), according to the manufacturer's instructions. Samples were subsequently processed using the Affymetrix GeneChip whole transcript sense target labelling assay and hybridized to the Affymetrix Exon 1.0 ST or U133 Plus 2.0 Arrays following the recommended Affymetrix protocols. Hybridized arrays were scanned on GeneChip Scanner 3000 and visually inspected for hybridization artefacts. The data was deposited in the GEO database under accession numbers GSE28365 and GSE30792 . Analysis of microarray data Exon Array data generated from fibroblast lines ( n =2), iPSC lines ( n =4) and neuralized iPSC lines ( n =8) were evaluated for uniform hybridization intensity, abnormal background signals and sample outliers using Affymetrix Expression Console (Affymetrix). All arrays were preprocessed using RMA quantile normalization with GC background correction in Partek's Genomics Suite v6.5 (Partek). Only probe sets containing a minimum of 3 probes, unique hybridization and designed against genes annotated within Entrez Gene ( http://www.ncbi.nlm.nih.gov/entrez/query.fcgi?db=gene ) as documented in the most recent Netaffx annotation file (HuEx-1_0-st-v2 Probeset Annotations, CSV Format, Release 31) were included in the analysis. Gene level summary signals were generated by calculating the median expression value of all probe sets annotated to a single gene. PCA, unsupervised hierarchical clustering, t -testing and gene expression scatterplot analyses were performed in Partek Genomics Suite v6.5 (Partek). GSEA was performed using GSEA v2.0.6 (Broad Institute) using gene set permutation and a triplication gene set, which was defined as all genes present within the triplication region (as identified on SNP array assessment) [40] . Following removal of batch effects, iPSC data analysed using Affymetrix U133 Plus 2.0 Arrays were compared via principal components analysis with the following data sets, all publicly available via the GEO database under accession codes: GSE16190 , GSE19902 , GSE22499 , GSE26451 , GSE7179 , GSE7879 , GSE8590 and GSE9440 . Accession codes: The SNP data generated in this study has been deposited in the GEO database under accession code GSE28366 . The microarray data generated in this study has been deposited in the GEO database under accession codes GSE28365 and GSE30792 . How to cite this article: Devine, M.J. et al . Parkinson's disease induced pluripotent stem cells with triplication of the α-synuclein locus. Nat. Commun. 2:440 doi: 10.1038/ncomms1453 (2011).